Hypoxia promotes stem cell phenotypes and poor prognosis through epigenetic regulation of DICER MicroRNAs are small regulatory RNAs that post transcriptionally control gene expression. Reduced expression of DICER, the enzyme involved in microRNA processing, is frequently observed in cancer and is associated with poor clinical outcome in various malignancies. Yet, the underlying mechanisms are not well understood. Here we identify tumour hypoxia as a regulator of DICER expression in large cohorts of breast cancer patients. We show that DICER expression is suppressed by hypoxia through an epigenetic mechanism that involves inhibition of oxygen-dependent H3K27me3 demethylases KDM6A/B and results in silencing of the DICER promoter. Subsequently, reduced miRNA processing leads to derepression of the miR-200 target ZEB1, stimulates the epithelial to mesenchymal transition and ultimately results in the acquisition of stem cell phenotypes in human mammary epithelial cells. Our study uncovers a previously unknown relationship between oxygen-sensitive epigenetic regulators, miRNA biogenesis and tumour stem cell phenotypes that may underlie poor outcome in breast cancer. Cancer mortality is largely attributable to distant metastasis. The mechanisms underlying the metastatic process are complex and are part of a series of events that ultimately result in the formation of macroscopic metastasis in distant organs from cells with tumour initiating or ‘stem cell’ properties [1] . Acquisition of stem cell and metastatic traits that enable this process, and the conditions in tumours that stimulate it, are poorly understood. However, many recent studies indicate that some tumour cells are able to transition from an epithelial to mesenchymal (EMT) phenotype through a process similar to that which occurs in development. Acquisition of the mesenchymal phenotype is associated with both increased tumour-initiating properties and the ability to form metastases in experimental models. However, in tumours this process requires some degree of plasticity, as formation of a tumour at a secondary metastatic site requires transition back to the epithelial cell state (mesenchymal to epithelial transition). Micro RNAs (miRNAs) are small regulatory RNAs that play an important role in normal development and in disease by regulating the expression of a vast number of target messenger RNAs [2] . miRNA biogenesis begins with transcription of long primary miRNAs (pri-miRNA) containing one or more hairpin structures that are processed by the nuclear endonuclease DROSHA, generating a 70-nucleotide stem loop known as the precursor miRNA (pre-miRNA). The pre-miRNA is exported to the cytoplasm by XPO5, and cleaved by DICER in a complex with TRBP2 to generate a ~22-nucleotide mature miRNA duplex. One strand is loaded into the RNA-induced silencing complex, which controls gene expression through sequence-specific interactions with target mRNAs causing their degradation or translational repression [3] . Several members of this miRNA biogenesis pathway have been identified as haplo-insufficient tumour suppressors, including DICER itself, XPO5 and TRBP2 (refs 4 , 5 , 6 , 7 , 8 , 9 , 10 ). Using a variety of mouse models, these studies indicate that partial suppression of miRNA biogenesis is sufficient to accelerate tumour development. Loss of one DICER allele in mouse models results in a reduction in overall levels of mature miRNA and increased lung and soft tissue sarcomas [4] , [5] . These studies extend earlier clinical findings, demonstrating that miRNA levels are frequently reduced in tumours [6] . It is not clear how a reduction in miRNA biogenesis promotes cancer and whether loss of one or more specific miRNAs underlies this effect. However, miRNA has been hypothesized to confer ‘robustness’ to biological processes including stabilizing differentiated cell states [11] . In patients, low levels of DICER in breast, ovarian and other cancers are associated with aggressive, invasive disease, distant recurrence and poor overall survival [12] , [13] , [14] . In several model systems, DICER repression has also been shown to stimulate metastasis [7] , [10] . In addition to monoallelic loss in cancer [5] , several mechanisms have been described as potential regulators of DICER including the transcription factors MITF [15] and Tap63 (ref. 10 ) and miR-103/107 (ref. 7 ). DICER expression has also been reported to be inhibited by hypoxia through an unknown mechanism [16] . Hypoxia is a common feature of tumours strongly associated with poor prognosis in multiple sites, including breast cancer [17] , [18] , [19] . Clinical studies show a strong association between hypoxia and distant metastasis or relapse [19] , [20] , [21] , [22] , [23] , [24] . Laboratory data support a direct role for hypoxia in driving metastasis, including in vivo studies with cell line-derived [25] , [26] , and more recently, patient-derived xenografts grown in the orthotopic site. Hypoxia has been suggested to promote stemness in both normal tissues and tumours [27] , [28] , [29] , [30] , [31] , [32] . However, the mechanisms driving this aggressive phenotype are poorly understood. In this study we have identified a new mechanism linking hypoxia, reduced miRNA biogenesis and acquisition of phenotypes associated with poor outcome. We show that tumour hypoxia is associated with reduced DICER expression in large cohorts of breast cancer patients and identify an epigenetic mechanism that suppresses DICER transcription through inhibition of oxygen-dependent H3K27me3 demethylases KDM6A/B. In breast cancer, reduced expression of DICER leads to a selective decrease in processing of the miR-200 family and consequently to derepression of ZEB1 and activation of the EMT and associated stem cell phenotypes. Reduced DICER expression in hypoxic human breast cancers Both experimental and clinical data have demonstrated a strong correlation between hypoxia and more aggressive disease, including phenotypes recently linked to DICER suppression, such as stemness [33] and metastasis [18] , [25] . We therefore examined the association between DICER expression, DICER copy number and hypoxia in breast cancer. We stratified breast cancer patients from two data sets (METABRIC [34] and The Cancer Genome Atlas (TCGA) [35] ) having normal DICER copy number by the amount of hypoxia as determined using the validated Winter hypoxia signature [36] ( Fig. 1a and Supplementary Fig. 1a ). The median RNA expression of 99 hypoxia associated genes in the Winter signature is an independent prognostic factor in head and neck squamous cell carcinoma and breast cancer series. In both data sets, patients with the largest hypoxic fraction exhibited the lowest DICER mRNA expression ( Fig. 1a and Supplementary Fig. 1a ). A significant inverse correlation between hypoxia and DICER expression was found for the TCGA, METABRIC, Harris and 14 out of 18 smaller breast cancer gene expression studies ( Fig. 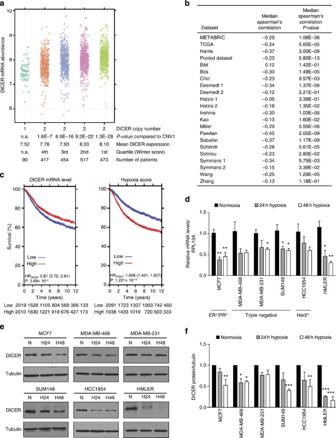Figure 1: Impaired DICER expression in hypoxic human breast cancers. (a) DICER mRNA abundance in breast cancer patients from METABRIC stratified byDICERcopy number and hypoxic fraction as determined with the Winter hypoxia metagene.P-values obtained with Wilcoxon rank sum test. (b) Inverse correlation between DICER mRNA abundance and hypoxia score.P-values obtained with Spearman’s correlation. (c) Kaplan–Meier survival curves for DICER and hypoxia in pooled breast cancer data set consisting of 19 studies. (d) RNA was extracted from indicated breast cancer cell lines exposed to 0.2% O2for 24 or 48 h and subjected to quantitative reverse transcriptase–PCR analysis of DICER with RPL13A as control (n≥3). Data represent mean±s.e.m.P-values obtained with one-way analysis of variance (ANOVA), Bonferroni’spost-hoctest. (e) Representative western blottings were performed with antibody against DICER and anti-tubulin as control. (f) Densitometric analysis of western blottings inewhere the intensity of the DICER bands were normalized for tubulin signal (n=3). Error bars represent s.e.m.P-values obtained with one-way ANOVA, Bonferroni’spost-hoctest. *P<0.05, **P<0.01, ***P<0.001. 1b and Supplementary Table 1 ). A pooled data set, consisting of 19 studies with long-term clinical follow-up, also demonstrated a highly significant ( P =5.80 × 10 −13 ) inverse correlation between DICER and hypoxia. Interestingly, in both the pooled and METABRIC data sets, low levels of DICER and high levels of hypoxia were associated with poor outcome ( Fig. 1c and Supplementary Figs 2 and 3 ). Notably, the reduction in DICER expression in the most hypoxic quartile was reduced to levels similar to that in the ~5% of tumours that had monoallelic loss of DICER . These data suggest that hypoxia is a key contributor to DICER expression and is responsible for reduced DICER levels in significantly more patients than genetic loss. We confirmed that hypoxia suppresses DICER at both the mRNA and protein level in a panel of breast cancer (MCF7, MDA-MB-468, MDA-MB-231, SUM149 and HCC1954), normal (MCF10A) or transformed (HMLER) mammary epithelial cell lines after exposure to oxygen levels commonly found in human tumours (<0.02 to 1.0% O 2 ) ( Fig. 1d–f and Supplementary Fig. 4 ). Hypoxic suppression varied from 26% to 74% at the mRNA level and 16% to 84% at the protein level over a period of 24–48 h of hypoxia. DICER repression in hypoxia was not associated with any particular breast cancer subtype in either the cell lines or in the breast cancer clinical data sets ( Supplementary Figs 2 and 3 , and Supplementary Table 1 ). Figure 1: Impaired DICER expression in hypoxic human breast cancers. ( a ) DICER mRNA abundance in breast cancer patients from METABRIC stratified by DICER copy number and hypoxic fraction as determined with the Winter hypoxia metagene. P -values obtained with Wilcoxon rank sum test. ( b ) Inverse correlation between DICER mRNA abundance and hypoxia score. P -values obtained with Spearman’s correlation. ( c ) Kaplan–Meier survival curves for DICER and hypoxia in pooled breast cancer data set consisting of 19 studies. ( d ) RNA was extracted from indicated breast cancer cell lines exposed to 0.2% O 2 for 24 or 48 h and subjected to quantitative reverse transcriptase–PCR analysis of DICER with RPL13A as control ( n ≥3). Data represent mean±s.e.m. P -values obtained with one-way analysis of variance (ANOVA), Bonferroni’s post-hoc test. ( e ) Representative western blottings were performed with antibody against DICER and anti-tubulin as control. ( f ) Densitometric analysis of western blottings in e where the intensity of the DICER bands were normalized for tubulin signal ( n =3). Error bars represent s.e.m. P -values obtained with one-way ANOVA, Bonferroni’s post-hoc test. * P <0.05, ** P <0.01, *** P <0.001. Full size image In addition to monoallelic loss in cancer, several mechanisms have been implicated in DICER regulation. These include the transcription factors MITF [15] and Tap63 (ref. 10 ), which induce DICER, miR-103/107, which repress DICER [7] , and a Von Hippel-Lindau (VHL)-dependent mechanism affecting DICER protein stability [16] . We examined each of these and found that none could explain suppression of DICER by hypoxia in breast cancer. Reporter constructs containing 2.5 kb of the DICER promoter (with or without mutations in the MITF E-box elements) showed no regulation by hypoxia ( Supplementary Fig. 5a,b ). Similarly, no increase in miR-103/107 and no decrease in DICER transcript or protein stability were observed during hypoxia ( Supplementary Fig. 5c–f ). We also observed no significant difference in DICER repression in cell lines isogenic for VHL ( Supplementary Fig. 5g ). Importantly, MITF, Tap63 and miR-103/107 also showed weak or no correlation with DICER expression in breast cancer patients in the TCGA and METABRIC data sets ( Supplementary Fig. 1b–h ). DICER is epigenetically regulated during hypoxia The lack of regulation of the DICER reporter construct ( Supplementary Fig. 5a,b ) during hypoxia was surprising. To directly test whether transcription of the endogenous DICER locus was affected, we measured changes in de novo transcription during hypoxia by pulse-labelling RNA. These experiments demonstrated that DICER transcription decreased 40% to 50% during hypoxia ( Fig. 2a ), whereas the HIF1 target gene carbonic anhydrase-9 ( CA9 ) increased 20-fold ( Supplementary Fig. 7a ). Transcriptional suppression of DICER was not dependent on known hypoxia response pathways, including either the HIF (hypoxia-inducible factor) pathway (as reported previously [16] ) or the PERK/ATF4 arm of the unfolded protein response ( Supplementary Fig. 6a–e ). DICER repression occurred normally in both HIF1α knockout cells and in multiple lines where HIF1α was depleted by RNA interference ( Supplementary Fig. 6a–c ). In addition, hypoxic downregulation of DICER did not affect HIF regulation in breast cancer cell lines, which has been previously reported in other cell types [16] ( Supplementary Fig. 6f ). 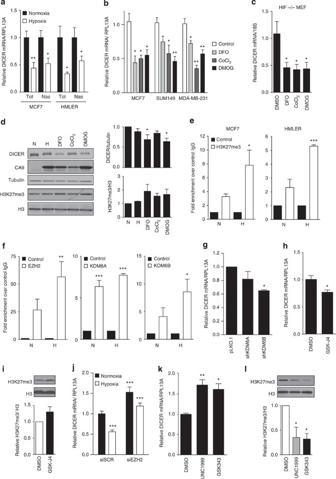Figure 2: Epigenetic silencing of DICER promoter in response to hypoxia. (a) Total (Tot) and nascent (Nas) DICER mRNA expression during hypoxia in MCF7 and HMLER cell lines was determined using quantitative reverse transcriptase–PCR (qRT–PCR) with RPL13A as control (n=4). (b) Indicated breast cancer cell lines (n=3) or (c) HIF1α-null mouse embryonic fibrobasts (MEFs) (n=4) were exposed to 500 μM iron chelator DFO, 250 μM antagonist CoCl2or 500 μM DMOG for 24 h. DICER mRNA expression was determined using qRT–PCR with RPL13A or 18S as control. (d) Western blot analysis of MCF7 cell extracts prepared after 24 h exposure to 0.2% O2, 500 μM DFO, 250 μM CoCl2or 500 μM DMOG with antibodies specific for DICER, CA9 and H3K27me3. Tubulin and H3 serve as respective loading controls. Representative blot (right) and densitometric analysis of western blottings from four independent experiments (left). (e) Validation of the enrichment in H3K27me at the DICER promoter was done using ChIP analysis of H3K27me3 mark in combination with qRT–PCR analysis in MCF7 and HMLER cells during normoxia (N) or hypoxia (H). Fold-enrichment shown over control IgG (n=3). (f) Enrichment of EZH2, KDM6A or KDM6B at the DICER promoter was done using ChIP analysis of each enzyme in combination with qRT–PCR analysis in MCF7 cells during normoxia (N) and hypoxia (H) (n=3). (g,h) qRT–PCR analysis of DICER expression with RPL13A as control in MCF7 cells (g) bearing shRNAs against KDM6A/B (n=3) or (h) treated with 10 μM KDM6A/B inhibitor GSK-J4 24 h (n=3). (i) Representative blot (top) and quantification of global H3K27me3 (bottom) after GSK-J4 treatment inh. DICER mRNA expression in MCF7 cells (j) transiently transfected with siRNA directed against EZH2 during aerobic and hypoxic conditions (n=4) or (k) treated with 5 μM EZH2 inhibitor UNC1999 or GSK343 for 48 h (n=3). (l) Representative western blotting (top) and quantification of global H3K27me3 levels (bottom) after EZH2 inhibition ink. Error bars represent s.e.m.P-values obtained with Student’st-test or one-way analysis of variance, Bonferroni’spost-hoctest. *P<0.05, **P<0.01, ***P<0.001. Figure 2: Epigenetic silencing of DICER promoter in response to hypoxia. ( a ) Total (Tot) and nascent (Nas) DICER mRNA expression during hypoxia in MCF7 and HMLER cell lines was determined using quantitative reverse transcriptase–PCR (qRT–PCR) with RPL13A as control ( n =4). ( b ) Indicated breast cancer cell lines ( n =3) or ( c ) HIF1α-null mouse embryonic fibrobasts (MEFs) ( n =4) were exposed to 500 μM iron chelator DFO, 250 μM antagonist CoCl 2 or 500 μM DMOG for 24 h. DICER mRNA expression was determined using qRT–PCR with RPL13A or 18S as control. ( d ) Western blot analysis of MCF7 cell extracts prepared after 24 h exposure to 0.2% O 2 , 500 μM DFO, 250 μM CoCl 2 or 500 μM DMOG with antibodies specific for DICER, CA9 and H3K27me3. Tubulin and H3 serve as respective loading controls. Representative blot (right) and densitometric analysis of western blottings from four independent experiments (left). ( e ) Validation of the enrichment in H3K27me at the DICER promoter was done using ChIP analysis of H3K27me3 mark in combination with qRT–PCR analysis in MCF7 and HMLER cells during normoxia (N) or hypoxia (H). Fold-enrichment shown over control IgG ( n =3). ( f ) Enrichment of EZH2, KDM6A or KDM6B at the DICER promoter was done using ChIP analysis of each enzyme in combination with qRT–PCR analysis in MCF7 cells during normoxia (N) and hypoxia (H) ( n =3). ( g , h ) qRT–PCR analysis of DICER expression with RPL13A as control in MCF7 cells ( g ) bearing shRNAs against KDM6A/B ( n =3) or ( h ) treated with 10 μM KDM6A/B inhibitor GSK-J4 24 h ( n =3). ( i ) Representative blot (top) and quantification of global H3K27me3 (bottom) after GSK-J4 treatment in h . DICER mRNA expression in MCF7 cells ( j ) transiently transfected with siRNA directed against EZH2 during aerobic and hypoxic conditions ( n =4) or ( k ) treated with 5 μM EZH2 inhibitor UNC1999 or GSK343 for 48 h ( n =3). ( l ) Representative western blotting (top) and quantification of global H3K27me3 levels (bottom) after EZH2 inhibition in k . Error bars represent s.e.m. P -values obtained with Student’s t -test or one-way analysis of variance, Bonferroni’s post-hoc test. * P <0.05, ** P <0.01, *** P <0.001. Full size image Although HIF1 was not required for DICER suppression during hypoxia, we found that agents that stabilize HIF by inhibiting the HIF prolyl-hydroxylases (EGLN1/2/3) did cause DICER suppression. Deferoxamine (DFO), cobalt chloride (CoCl 2 ) and dimethyloxalylglycine (DMOG) at concentrations sufficient to activate transcription of HIF1 target genes (for example, CA9 — Supplementary Fig. 7b ) all resulted in a significant reduction in DICER at the mRNA and protein level ( Fig. 2b,d ). DFO and CoCl 2 stabilize HIF by chelating or competing with iron [Fe(II)], whereas DMOG does so by competitive inhibition of 2-oxogluterate, which in addition to oxygen, are required co-factors for the HIF prolyl-hydroxylases that mediate HIF stability. However, similar to hypoxia, treatment with DFO, CoCl 2 and DMOG also caused DICER repression in HIF1α knockout cells ( Fig. 2c ). As hypoxia, DFO, CoCl 2 and DMOG all influenced DICER expression in a HIF1α-independent manner, we hypothesized that DICER was regulated through inhibition of alternative iron, oxygen and 2-oxogluterate-dependent enzymes, such as the Jumonji-domain containing hydroxylases KDM6A and KDM6B [37] that regulate epigenetic silencing through removal of repressive histone 3 lysine 27 trimethylation (H3K27me3) marks [38] . Indeed, inhibition of all three required cofactors of the KDM6A/B enzymes by hypoxia, DFO, CoCl 2 and DMOG resulted in an increase in total H3K27me3 in multiple cell types ( Fig. 2d and Supplementary Fig. 7c ). More importantly, H3K27me3 chromatin immunoprecipitation followed by sequencing (ChIP-seq) demonstrated that hypoxic exposure for as short as 8 h led to an increase in repressive H3K27me3 marks in the DICER promoter region ( Supplementary Fig. 7d ). Enrichment in H3K27me3 at the DICER promoter during hypoxia was confirmed using conventional ChIP–quantitative PCR (qPCR) in MCF7 (eightfold enrichment versus hypoxic IgG control) and HMLER (fivefold enrichment versus hypoxic IgG control) cell lines ( Fig. 2e ). In both cell lines, this translated into an approximate doubling of H3K27me3 as compared with levels under normoxia. Furthermore, ChIP–qPCR analysis using specific antibodies against the H3K27 methyltransferase EZH2 (writer) and the oxygen-dependent H3K27me3 demethylases KDM6A and KDM6B (erasers) revealed significant enrichment over IgG controls at the DICER promoter for each respective enzyme, with no significant difference in enrichment between normoxic and hypoxic conditions ( Fig. 2f ). Consistent with a role for epigenetic regulation of DICER, knockdown of KDM6A or KDM6B resulted in reduced DICER expression ( Fig. 2g and Supplementary Fig. 7e–g ). Similarly, inhibition of KDM6A/B with the inhibitor GSK-J4 at concentrations that increased overall levels of H3K27me3 by 1.3-fold caused a 23% and 50% decrease in DICER expression in MCF7 and HMLER cells, respectively ( Fig. 2h,i and Supplementary Fig. 7h,i ) without affecting HIF activity ( Supplementary Fig. 7h ). Conversely, knockdown of EZH2 resulted in a significant increase in DICER expression and was able to largely prevent DICER repression during hypoxia ( Fig. 2j and Supplementary Fig. 7j ). Similarly, inhibition of EZH2 using UNC1999 and GSK343 at levels that caused decreases in global H3K27me3 levels by 50%–70% ( Fig. 2l and Supplementary Fig. 7k ) also increased DICER to levels comparable with EZH2 knockdown ( Fig. 2k and Supplementary Fig. 7l ). Together, these data indicate that basal expression of DICER is regulated by dynamic and opposing activities of KDM6A/B and EZH2, which are both constitutively present at the DICER locus, and that suppression of KDM6A/B activity under hypoxia is sufficient to increase H3K27me3 in an EZH2-dependent manner and suppress DICER transcription. Hypoxia causes an miRNA processing defect To examine the consequences of DICER suppression, we created MCF7 and HMLER breast cancer cell lines with stable knockdown of DICER and assessed changes in levels of mature miRNA. Suppression of DICER to ~30% resulted in a widespread reduction in mature miRNA for the majority of miRNA species ( Fig. 3a,b and Supplementary Fig. 8a ). Hypoxia also led to an analogous impairment in the processing of exogenously introduced short hairpin (shRNA) ( Supplementary Fig. 8b ). Short interfering RNA (siRNA) and shRNA targeting HIF1α showed similar efficiency under aerobic conditions, but under hypoxia HIF1α shRNA, which requires DICER processing, was significantly less efficient. Under hypoxia, HIF1α siRNA reduced the HIF target gene CA9 by ~50%, whereas HIF1α shRNA failed to prevent CA9 induction. 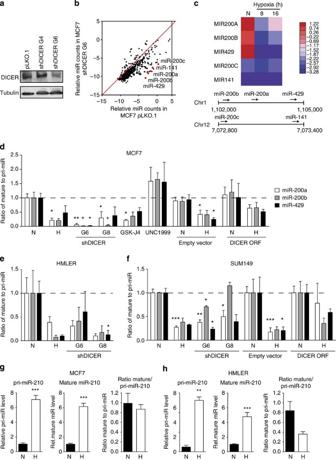Figure 3: Impaired miRNA processing in hypoxic cells. (a) MCF7 cells were transduced with lentiviral shRNA constructs directed at DICER. Cell extracts from MCF7 cells bearing empty vector pLKO.1, non-functional shDICER_G4 or functional shDICER_G6 were subjected to western blot analysis using a DICER-specific antibody. Tubulin served as loading control. (b) Total RNA was extracted from MCF7 pLKO.1 or shDICER_G6. miRNA levels were determined by Nanostring technology (n=3). (c) MCF7 cells exposed to hypoxia (<0.02% O2) for 16 h were used for total RNA isolation and subsequently subjected to deep-sequence analysis of miRNA content. Heat map of the miR-200 family in MCF7 during hypoxia is shown. Bottom panel shows schematic representation of the genomic organization of the miR-200 family. (d) The ratio of mature miRNA to pri-miRNA for miR-200a, b and 429 in MCF7 cells after hypoxia, DICER knockdown (shRNA G6 and G8), KDM6 inhibitor GSK-J4 (10 μM), EZH2 inhibitor UNC1999 (5 μM) and DICER overexpression. Mature and pri-miRNA levels were determined by quantitative reverse transcriptase–PCR (qRT–PCR). Similar experiments were performed in (e) HMLER and (f) SUM149 cells. (g,h) Processing of hypoxia-inducible miR-210 was assessed as described indfor (g) MCF7 and (h) HMLER cells. Expression levels of mature and pri-miRNAs for the miR-210 family was determined by qRT–PCR. N, normoxia; H, hypoxia. Data ind–hrepresent mean ratios (n=3)±s.e.m.P-values obtained with Student’st-test. *P<0.05, **P<0.01, ***P<0.001. Figure 3: Impaired miRNA processing in hypoxic cells. ( a ) MCF7 cells were transduced with lentiviral shRNA constructs directed at DICER. Cell extracts from MCF7 cells bearing empty vector pLKO.1, non-functional shDICER_G4 or functional shDICER_G6 were subjected to western blot analysis using a DICER-specific antibody. Tubulin served as loading control. ( b ) Total RNA was extracted from MCF7 pLKO.1 or shDICER_G6. miRNA levels were determined by Nanostring technology ( n =3). ( c ) MCF7 cells exposed to hypoxia (<0.02% O 2 ) for 16 h were used for total RNA isolation and subsequently subjected to deep-sequence analysis of miRNA content. Heat map of the miR-200 family in MCF7 during hypoxia is shown. Bottom panel shows schematic representation of the genomic organization of the miR-200 family. ( d ) The ratio of mature miRNA to pri-miRNA for miR-200a, b and 429 in MCF7 cells after hypoxia, DICER knockdown (shRNA G6 and G8), KDM6 inhibitor GSK-J4 (10 μM), EZH2 inhibitor UNC1999 (5 μM) and DICER overexpression. Mature and pri-miRNA levels were determined by quantitative reverse transcriptase–PCR (qRT–PCR). Similar experiments were performed in ( e ) HMLER and ( f ) SUM149 cells. ( g , h ) Processing of hypoxia-inducible miR-210 was assessed as described in d for ( g ) MCF7 and ( h ) HMLER cells. Expression levels of mature and pri-miRNAs for the miR-210 family was determined by qRT–PCR. N, normoxia; H, hypoxia. Data in d – h represent mean ratios ( n =3)±s.e.m. P -values obtained with Student’s t -test. * P <0.05, ** P <0.01, *** P <0.001. Full size image Sensitivity to DICER knockdown varied among different miRNA and the five members of the miR-200 family (miR-200a, miR-200b, miR-429, miR-200c and miR-141) were among the most strongly repressed in both lines ( Fig. 3b and Supplementary Fig. 8a ). Similarly, the miR-200a/b/429 cluster was among the most strongly repressed miRNAs in response to hypoxia ( Fig. 3c ). We confirmed that both hypoxia and DICER knockdown led to a substantial defect in the processing of miR-200 family precursors (pri-miRNAs) into mature miRNAs. The ratio of mature to pri-miRNA, an indicator of DICER activity, dropped substantially in response to both DICER knockdown and hypoxia in MCF7, HMLER and SUM149 cells ( Fig. 3d–f and Supplementary Fig. 8c ). Furthermore, the reduction in DICER caused by inhibition of KDM6A/B using GSK-J4 also resulted in a decrease in miR-200a/b/429 processing similar to that during hypoxia or DICER knockdown ( Fig. 3d ). Conversely, inhibition of EZH2 using UNC1999, which increased DICER expression, increased miR-200a/b/429 processing ( Fig. 3d ). Importantly, transient overexpression of DICER during hypoxia increased miR-200a/b/429 processing to near basal levels, demonstrating that these effects on miRNA processing under hypoxia are due to its effects on DICER ( Fig. 3d,f and Supplementary Fig. 8d ). Despite the defect in miRNA processing caused by DICER repression, some mature miRNAs increased during hypoxia, including the widely reported hypoxia-inducible miR-210. However, in this case the increase is due entirely to a transcriptional effect ( Supplementary Fig. 8e,f and Fig. 3g,h ). The processing of miR-210 mediated by DICER is reduced under hypoxia, but this effect is smaller than the overall transcriptional increase, resulting in increased mature levels of the miRNA. Hypoxia stimulates EMT and CSC associated properties The miR-200 family is implicated in regulation of the ZEB1 and ZEB2 transcription factors, which repress E-cadherin and stimulate the EMT [39] . DICER knockdown has previously been implicated in promoting the EMT and metastasis through the miR-200 family [7] , and miR-200b repression and ZEB1 induction during hypoxia has been reported [40] , [41] . We hypothesized that DICER suppression during hypoxia may similarly regulate the EMT and perhaps underlie the known association of tumour hypoxia with metastasis, stemness and aggressive disease. Indeed, DICER repression in response to hypoxia or knockdown resulted in enhanced expression of ZEB1, loss of epithelial marker expression (E-cadherin) and increased expression of mesenchymal markers (N-cadherin and Vimentin) ( Fig. 4a–c ). The transcription factor TWIST, previously implicated in hypoxia-induced EMT and metastasis [42] , remained unchanged, as did the transcription factor SNAIL ( Supplementary Fig. 9a,b ). The hypoxia- and DICER knockdown-induced EMT is mechanistically distinct from the classical EMT inducer transforming growth factor-β1 (TGFβ1), which was associated with increased expression of TWIST and SNAIL, but caused no change in DICER expression or miRNA biogenesis ( Supplementary Fig. 9c–e ). 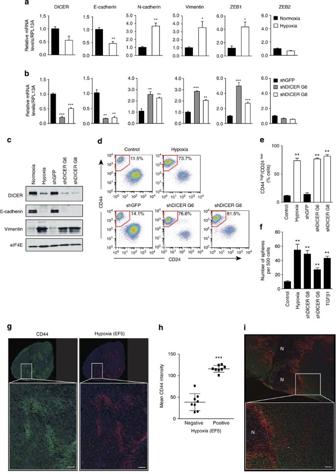Figure 4: DICER repression promotes cancer stem cell-associated phenotypes by reduced miR-200 expression during hypoxia. (a) HMLER cells were grown for 7 days under 1% O2. RNA was extracted and used to determine DICER mRNA levels by quantitative reverse transcriptase–PCR analysis. Expression of epithelial and mesenchymal-associated genes was assessed simultaneously. RPL13A served as control (n=3). (b) Similar analysis as inawas performed on HMLER cells transduced with two independent shRNA constructs targeting DICER (n=3). (c) HMLER protein extracts were subjected to western blot analysis of DICER, E-cadherin, Vimentin and eIF4E as loading control. (d) Representative FACS analysis of HMLER cells using antibodies specific for CD44 and CD24. (e) Quantification of the percentage of cells with CD44highCD24lowfor three independent experiments. (f) Sphere formation assay, number of spheres formed per 500 cells plotted (n=3). (g) Representative image of whole tumour (top) and 25 × region (bottom) of CD44 (green), EF5 (red) and DAPI (blue) staining in HMLER orthotopic xenograft. (h) Mean CD44 intensity in hypoxic (EF5 negative) versus non-hypoxic (EF5 positive) tumour regions of HMLER xenografts (n=8 mice). (i) Representative image of whole tumour (top) and 25 × region (bottom) of H3K27me3 (green), EF5 (red) and DAPI (blue) staining in HMLER orthotopic xenograft. N indicates regions of tumour necrosis. Scale bar, 100 μm. Error bars represent s.e.m.P-values obtained with Student’st-test or one-way analysis of variance, Bonferroni’spost-hoctest. *P<0.05, **P<0.01, ***P<0.001. Figure 4: DICER repression promotes cancer stem cell-associated phenotypes by reduced miR-200 expression during hypoxia. ( a ) HMLER cells were grown for 7 days under 1% O 2 . RNA was extracted and used to determine DICER mRNA levels by quantitative reverse transcriptase–PCR analysis. Expression of epithelial and mesenchymal-associated genes was assessed simultaneously. RPL13A served as control ( n =3). ( b ) Similar analysis as in a was performed on HMLER cells transduced with two independent shRNA constructs targeting DICER ( n =3). ( c ) HMLER protein extracts were subjected to western blot analysis of DICER, E-cadherin, Vimentin and eIF4E as loading control. ( d ) Representative FACS analysis of HMLER cells using antibodies specific for CD44 and CD24. ( e ) Quantification of the percentage of cells with CD44 high CD24 low for three independent experiments. ( f ) Sphere formation assay, number of spheres formed per 500 cells plotted ( n =3). ( g ) Representative image of whole tumour (top) and 25 × region (bottom) of CD44 (green), EF5 (red) and DAPI (blue) staining in HMLER orthotopic xenograft. ( h ) Mean CD44 intensity in hypoxic (EF5 negative) versus non-hypoxic (EF5 positive) tumour regions of HMLER xenografts ( n =8 mice). ( i ) Representative image of whole tumour (top) and 25 × region (bottom) of H3K27me3 (green), EF5 (red) and DAPI (blue) staining in HMLER orthotopic xenograft. N indicates regions of tumour necrosis. Scale bar, 100 μm. Error bars represent s.e.m. P -values obtained with Student’s t -test or one-way analysis of variance, Bonferroni’s post-hoc test. * P <0.05, ** P <0.01, *** P <0.001. Full size image In breast cancer, the EMT has been linked to acquisition of stem cell phenotypes, including expression of cell surface antigens associated with human breast stem cells (CD44 high CD24 low ), increased mammosphere formation and increased tumour initiation capacity [43] , [44] , [45] . In HMLER cells, hypoxic exposure led to an increase in the frequency of CD44 high CD24 low cells from 11.5% to 73.7% ( Fig. 4d,e ), comparable to levels observed following exposure to TGFβ1 ( Supplementary Fig. 9e ) or reported following forced exposure of SNAIL or TWIST [43] . A similar increase in the fraction of CD44 high CD24 low cells occurred following DICER knockdown alone (76.6% and 81.5% versus 14.1%) ( Fig. 4d,e ). Both hypoxic exposure and DICER knockdown resulted in a greater than fivefold increase in mammosphere formation similar to that observed following TGFβ1 exposure ( Fig. 4f ). Importantly, hypoxia is similarly able to influence H3K27me3, DICER, EMT and stem cell phenotypes in vivo . We established HMLER xenografts and examined the spatial relationship between hypoxia, H3K27me3 and CD44 using multi-fluorescence immunohistochemistry. As shown in Fig. 4g,h , tumour hypoxia in vivo (as assessed by EF5) is strongly associated with increased expression of the stem cell marker CD44 ( Fig. 4g,h ). Hypoxic tumour areas also show increased overall levels of H3K27me3, with discernable gradients in expression away from hypoxic areas ( Fig. 4i ). Furthermore, we assessed DICER, ZEB1 and E-cadherin expression in vivo using a panel of breast cancer xenografts and found that DICER and E-cadherin were inversely correlated with the endogenous hypoxia marker CA9, whereas ZEB1 showed a positive correlation with CA9 ( Supplementary Fig. 9f ). Finally, we tested directly if hypoxia- and DICER knockdown-induced EMT and acquisition of stem cell phenotypes is dependent on loss of mature miR-200 levels. DICER overexpression during hypoxia, which rescued the defect in miR-200 processing ( Fig. 3d ), also prevented increased expression of ZEB1 ( Supplementary Fig. 9g ). Furthermore, overexpression of miR-200b alone prevented increased expression of ZEB1 and loss of E-cadherin during hypoxia, without affecting DICER repression and the defect in miRNA biogenesis ( Fig. 5a,b ). miR-200b overexpression during hypoxia also prevented the increase in the CD44 high CD24 low population and mammosphere formation ( Fig. 5c–e ). Together, these demonstrate that hypoxic suppression of DICER causes an EMT-driven acquisition of stem cell properties in breast cancer through a reduction in the biogenesis of mature miR-200 family members ( Fig. 5f ). 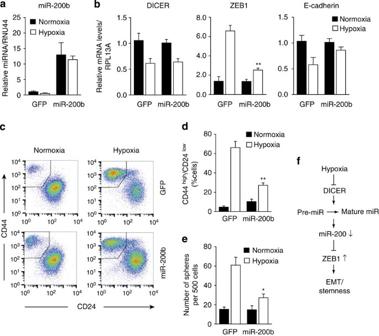Figure 5: Hypoxia stimulates cancer stem cell-associated phenotypes in a miR-200b-dependent manner. HMLER cells overexpressing miR-200b or green fluorescent protein (GFP) (n=3) grown for 7 days under 1% O2or control conditions. (a,b) quantitative reverse transcriptase–PCR analysis was performed to measure (a) mature miR-200b levels and (b) DICER, ZEB1 and E-cadherin mRNA levels where RPL13A served as control (n=3). (c) Representative FACS analysis using antibodies specific for CD44 and CD24. (d) Quantification of the percentage of cells with CD44highCD24lowfor three independent experiments. (e) Sphere formation assay, number spheres formed per 500 cells plotted (n=3). (f) Model of hypoxia-mediated EMT and stemness. Error bars represent s.e.m.P-values obtained with Student’st-test. *P<0.05, **P<0.01. Figure 5: Hypoxia stimulates cancer stem cell-associated phenotypes in a miR-200b-dependent manner. HMLER cells overexpressing miR-200b or green fluorescent protein (GFP) ( n =3) grown for 7 days under 1% O 2 or control conditions. ( a , b ) quantitative reverse transcriptase–PCR analysis was performed to measure ( a ) mature miR-200b levels and ( b ) DICER, ZEB1 and E-cadherin mRNA levels where RPL13A served as control ( n =3). ( c ) Representative FACS analysis using antibodies specific for CD44 and CD24. ( d ) Quantification of the percentage of cells with CD44 high CD24 low for three independent experiments. ( e ) Sphere formation assay, number spheres formed per 500 cells plotted ( n =3). ( f ) Model of hypoxia-mediated EMT and stemness. Error bars represent s.e.m. P -values obtained with Student’s t -test. * P <0.05, ** P <0.01. Full size image Our study demonstrates that hypoxia in the tumour microenvironment is a contributor to DICER expression and repression of miRNA biogenesis. In large independent cohorts of breast cancer patients, the association between hypoxia and DICER is stronger than any previously reported regulator of DICER, and the number of patients affected by this mechanism exceeds those harbouring monoallelic loss. This analysis also indicates that DICER suppression may underlie part of the known association of hypoxia with metastasis and poor outcome, although hypoxia remains a better discriminator than DICER in breast cancer patients. This is perhaps not surprising given that hypoxia influences other important biological processes, including angiogenesis, altered metabolism and chromosomal instability. The changes in histone methylation and DICER expression are relatively small (approximately twofold) in response to hypoxia or inhibition of EZH2 and KDM6A/B. Previous studies unambiguously identified DICER as a haploinsufficient tumour suppressor and an important driver of tumorigenesis under conditions of <50% repression [4] , [5] . Our study is consistent with these earlier reports and demonstrates that relatively small changes in DICER expression during hypoxia underlie functional changes in miRNA biogenesis, EMT and properties associated with stemness. Interestingly, Rupaimoole et al . have demonstrated that hypoxia causes additional suppression of miRNA biogenesis through silencing of DROSHA [46] and that the combined defect in miRNA biogenesis resulting from DICER and DROSHA suppression leads to increased metastasis in ovarian cancer. The coordinated suppression of these two key enzymes required for miRNA biogenesis as well as hypoxia-dependent suppression of AGO2 (ref. 47 ) suggests a particularly important and broad role for oxygen in the regulation of miRNA levels. The consequences of such regulation are likely to be different in specific tissues and cancer types, depending on the expression of different miRNAs. In breast cancer, we show that selective sensitivity of the miR-200 family to loss of DICER plays a dominant role in regulation of EMT and cancer stem cell phenotypes, which may underlie the known association of hypoxia with aggressive disease in breast and other cancer types [12] , [13] , [14] , [17] , [18] . Previous studies have reported multiple mechanisms of DICER regulation, which can occur at the level of transcription through MITF [15] and Tap63 (ref. 10 ), mRNA stability through miR-103/107, as well as at the protein level in a VHL-dependent manner [16] . Our study reveals that DICER transcription is also regulated dynamically by acquisition or loss of the repressive H3K27me3 polycomb mark that is typically associated with gene silencing [38] . This mark is also found on promoters of so-called ‘poised’ genes expressed at low levels in embryonic stem cells where it is often associated with co-occurrence of the activating H3K4 mark [48] . Several previous studies have indicated that the balance between writing (EZH2) and erasing (KDM6A/B) H3K27me3 marks within the genome can play an important role in cancer [49] , [50] . This is supported by the finding that EZH2 is frequently overexpressed or activated in cancer [51] , [52] , [53] , and associated with increased metastasis [54] . Conversely, the H3K27me3 demethylase KDM6A is frequently mutated in human cancers [55] , [56] and KDM6B expression is decreased in subsets of human cancers [57] , [58] . Our study identifies DICER as an important integrator of EZH2 methyltransferase and KDM6A/B demethylase activity. We showed that EZH2 and KDM6A/B are present at the DICER locus, and that inhibition of these enzymes can cause acute changes in the levels of H3K27me3, DICER expression and DICER activity. The hydroxylase activity of KDM6A/B requires molecular oxygen, 2-oxogluterate and Fe(II) to demethylate H3K27me3. Correspondingly, we found that hypoxia, or depletion/competition of the other co-factors with DFO, CoCl 2 or DMOG, all suppress DICER. To our knowledge, this is the first such example of a gene whose expression is dynamically regulated at the epigenetic level by the availability of metabolic enzymatic co-factors. As the basal levels of H3K27me3 are influenced by both EZH2 and KDM6A/B activities, we expect that additional metabolic co-factors that regulate their activity including methyl donation (EZH2) or 2-oxogluterate (KDM6A/B) will similarly influence DICER H3K27me3 levels and its expression. In contrast to genetic alteration of EZH2 and/or KDM6A/B, hypoxia-driven changes in the epigenetic state of DICER enables transient changes in cell phenotype in response to the local tumour microenvironment. In breast cancer, our findings demonstrate that suppression of DICER during hypoxia is sufficient to reduce miR-200 levels and enable cells to undergo an EMT and acquire stem cell properties. The fact that this occurs at the epigenetic level in an EZH2-dependent manner is consistent with a recent report that implicates EZH2 in controlling the EMT through epigenetic reprogramming [59] , but provides a potential mechanism for cells to retain plasticity and restore DICER and miR-200 levels when oxygen becomes available. Cancer cells need to undergo the reverse process, mesenchymal to epithelial transition, to ensure successful colonization and metastatic outgrowth [60] , [61] . We speculate that the clinical importance of hypoxia in driving metastasis and poor outcome is linked to this ability to transiently influence cell phenotype via DICER expression and miRNA biogenesis. Finally, our results provide new potential therapeutic opportunities for targeting hypoxia and its influence on poor outcome in cancer. Hypoxia has been demonstrated to influence patient outcome, both through its ability to promote metastatic growth of disseminated stem cells and for regrowth of tumours following treatment. Hypoxic cells are intrinsically resistant to radiation and other forms of chemotherapy and small numbers of these cells can ‘re-seed’ the tumour, enabling regrowth following therapy. Hypoxic tumour cells also arise as a consequence of treatment with anti-angiogenic agents and can contribute to tumour regrowth post therapy [62] . Consequently, the ability of hypoxic cells to stimulate tumour initiation—either in naive metastases or following therapy of primary tumours—is considered to play a large role in treatment outcome. It may be possible to interfere with the epigenetic regulation of DICER during hypoxia and/or its influence on the expression of key miRNAs that promote these adverse clinical effects. Recent potent, orally available inhibitors of EZH2 have been reported [63] , [64] and our results suggest that treatment with these agents induce DICER expression. Alternatively, an siRNA and/or miRNA strategy that does not rely on Drosha/Dicer processing and is not compromised within the tumour microenvironment could be applied. Effective delivery of siRNA and/or miRNA in vivo has improved remarkably and pre-clinical studies have demonstrated the potential of miR-200b delivery in breast, ovarian and other orthotopic models [65] . Data set analyses Retrieval and processing of breast cancer data sets . Preprocessing of raw mRNA abundance data sets was performed in R statistical environment (v2.14.1). Raw affymetrix-based data (PMIDs: 16273092, 17545524, 16141321, 16280042, 16478745, 18498629, 17157792, 19421193, 20098429, 20064235, 20490655, 20697068, 18821012, 18593943, 15721472, 21501481, 17079448, 21422418 and 21558518) were normalized using RMA (robust multi-array average) algorithm [66] (R package: affy v1.32.1). ProbeSet annotation to Entrez Gene IDs was performed using custom CDFs [67] (R packages: hgu133ahsentrezgcdf v15.0.0, hgu133bhsentrezgcdf v15.0.0, hgu133plus2hsentrezgcdf v15.0.0, hthgu133ahsentrezgcdf v15.0.0 and hgu95av2hsentrezgcdf v15.0.0 for affymetrix-based breast cancer data sets). The METABRIC breast cancer data set was preprocessed, summarized and quantile-normalized from the raw expression files generated by Illumina BeadStudio (R packages: beadarray v2.4.2 and illuminaHuman v3.db_1.12.2). Raw data files were downloaded from European genome-phenome archive (EGA) (Study ID: EGAS00000000083). Data files of one sample were not available at the time of this analysis and were therefore excluded. All data sets were normalized independently. Preprocessed segmented genome copy number aberration (CNA) data from the METABRIC cohort was downloaded from EGA. Preprocessed mRNA abundance data from TCGA were downloaded from cBioPortal for Cancer Genomics of Memorial Sloan-Kettering Cancer Center http://www.cbioportal.org/public-portal/ on 6 November 2012. Level 4 processed CNA data from TCGA were downloaded from GISTIC2 from the Broad Institute at http://gdac.broadinstitute.org/runs/analyses__2012_09_13/reports/cancer/BRCA/copynumber/gistic2/nozzle.html Discrete amplification and deletion calls for each sample based on the obtained CNA data were tabulated. For both mRNA abundance and CNA data, patient clinical information were obtained online from the original publication [35] . Calculation of Winter signature scores . For each gene in the Winter signature, each patient in a given cohort was assigned an initial score of either +1 or −1 as follows: a patient was assigned +1 if her expression of that gene exceeded the median expression of that gene in that complete cohort. Otherwise, the patient was assigned −1 for that gene. For each patient in a given cohort, the +1’s and −1’s obtained as described above over all genes in the Winter signature were summed and the resulting sum was the Winter signature score for that patient in that cohort. mRNA abundance correlation of Dicer with MITF or TP63 . For each of the Metabric (Training and Validation datasets combined) and TCGA breast cancer mRNA abundance data sets, a scatter plot was generated of the Dicer mRNA abundance against that of MITF. Pearson’s product–moment correlation coefficient of the mRNA abundance of the two genes was computed and its P -value, based on the two-sided t -test for the Pearson’s product–moment correlation, was computed. This analysis was repeated for the correlation of Dicer mRNA abundance and TP63 mRNA abundance. Comparison of Dicer mRNA abundance and Winter signature . For each of the Metabric (Training and Validation datasets combined) and TCGA breast cancer data sets, only patients with no Dicer copy number variation and those with monoallelic Dicer loss were retained. These retained patients were then divided into five groups as follows: those with monoallelic Dicer loss formed one group, and those with no Dicer copy number variation were ordered by their Winter signature scores and divided into four quarters, with the first quarter comprising patients with the lowest Winter signature scores, while the fourth represents those with highest Winter signature scores. A strip plot was generated to visualize the differences in Dicer mRNA abundance levels among these five groups. The Dicer mRNA abundance of patients in each of the four quarters of the group with no Dicer copy number variation was compared against the group with monoallelic Dicer loss, by computing the P -value based on the Wilcoxon rank sum test. Comparison of miR-103/107 expression and Winter signature . Analyses were carried out in R statistical environment (version 3.0.1) ( http:///www.r-project.org/ ). All tests were two-sided and considered statistically significant at the 0.05 level. Clinical and miRNA expression were downloaded from the Cancer Genome Atlas Project (TCGA) available through the associated files of the paper: ‘Comprehensive molecular portraits of human breast tumors, Nature , 27 September 2012’ ( https://tcga-data.nci.nih.gov/docs/publications/brca_2012/ ). We also downloaded Level 3 (RNASeqV2) genes profiles for Breast Invasive Carcinoma from TCGA Data Portal: https://tcga-data.nci.nih.gov/tcga/ . A hypoxia score was assigned to each TCGA sample based on the Winter hypoxia metagene signature and following the previously reported methodology [68] . The Shapiro–Wilk test was applied to verify whether the data follows a normal distribution. Accordingly, an analysis of variance test with Tukey post-hoc test was applied to assess the relationship between miR-103 and Winter hypoxia score, whereas a non-parametric test Kruskal–Wallis test with Nemenyi post-hoc test was applied to assess the relationship between miR-107 expression and Winter hypoxia score. Cell culture and treatment The following cell lines were obtained from ATCC and grown according to provided subculturing instructions: MCF7, MDA-MB-468, MDA-MB-231, T47D, U373, HCT116, Hela, ME180 and SiHa. HCC1954 and SUM149 cell lines were provided as a gift by Dr Benjamin Neel (Princess Margaret Cancer Centre). HCC1954 cells were grown in RPMI medium supplemented with 10% fetal bovine serum (FBS) and SUM149 cells were grown in Ham’s F12 medium supplemented with 5% FBS, insulin (5 μg ml −1 ), hydrocortisone (1 μg ml −1 ) and 10 mM Hepes (pH 7.4). HMLER cells were a gift from Dr Robert Weinberg (MIT) and were grown as previously described [69] . MCF10A cells were provided by Dr Senthil Muthuswamy (Princess Margaret Cancer Centre) and were grown in DMEM/F12 (Gibco BRL) supplemented with 5% donor horse serum, 20 ng ml −1 epidermal growth factor, 10 μg ml −1 insulin, 1 ng ml −1 cholera toxin, 100 μg ml −1 hydrocortisone, 50 μg ml −1 penicillin and 50 μg ml −1 streptomycin. Wild type and HIF1α−/− mouse embryonic fibrobasts, RCC4 and RCC4+pVHL were grown in DMEM medium supplemented with 10% FBS. All cell lines were routinely tested to confirm the absence of Mycoplasma . For hypoxic exposure, cells were transferred into a HypOxygen H35 workstation. The atmosphere in the chamber consisted of 5% H 2 , 5% CO 2 , the desired % O 2 and residual N 2 . For protein stability experiments, MCF7 cells were exposed to 100 μg ml −1 cycloheximide (Sigma) for 0, 2, 4 or 8 h of normoxia or 0.2% O 2 hypoxia. For exposure to stress-inducing agents, indicated cell lines were grown for 24 h in 250 μM CoCl 2 , 500 μM DFO or 500 μM DMOG. For inhibition of KDM6A/B activity, MCF7 and HMLER cells were grown for 24 h in GSK-J4 at indicated concentrations. For inhibition of EZH2 activity, MCF7 and HMLER cells were grown for 48–72 h in UNC1999 or GSK343 at indicated concentrations. For exposure to TGFβ1, HMLER cells were cultured in standard growth medium with the addition of 5% FBS and treated with 2.5 ng ml −1 TGFβ1 for 12 days. RNA extraction and quantitative reverse–transcription PCR RNA was isolated using TRI reagent (Sigma) and samples were reverse transcribed using qScript cDNA SuperMix (Quantas). Quantitative real-time PCR was performed on an Eppendorf Realplex [2] mastercycler using SYBR green (Quantas). Specific primers used are listed in Supplementary Table 2 . For determination of DICER mRNA half-life, cells were treated with 5 μg ml −1 actinomycin D (Sigma) for the indicated times. De novo RNA synthesis was measured using the Click-iT Nascent RNA Capture Kit (Molecular Probes). Briefly, MCF7 and HMLER cells were pulse labelled with 0.2 mM 5-ethynyl Uridine for 1 h during aerobic conditions or 24 h hypoxia (0.2% O 2 ) after which RNA was isolated as described above. Nascent RNA was captured using magnetic streptavidin beads, reverse transcribed and analysed by quantitative real-time PCR. For determination of pri-miRNA and mature miRNA levels, the following assays from Applied Biosystems were used: pri-miR200a (Hs03303376_pri), pri-miR200b (Hs03303027_pri), pri-miR429 (Hs03303727_pri), pri-miR200c (Hs03303157_pri), pri-miR141 (Hs03303157_pri), pri-miR210 (Hs03302948_pri), hsa-miR200a (000502), hsa-miR200b (002251), hsa-miR429 (001024), hsa-miR200c (002300), miR141 (002145), hsa-miR103 (000439), hsa-miR107 (000443), hsa-miR210 (000512), RNU44 (001094) and RNU48 (001006). Western blot analysis Cells were washed twice with cold PBS and scraped in 50 mM Tris HCl pH 8.0, 150 mM NaCl, 1% NP-40, 0.5% sodium deoxycholate and 0.1% SDS supplemented with protease and phosphatase inhibitors (Roche). After centrifugation at 10,000 g , supernatants were boiled in Laemmli buffer for 10 min and proteins were resolved by SDS–PAGE. Proteins were subsequently transferred onto polyvinylidene difluoride membrane and blocked for 1 h in TBS containing 0.05% Tween 20 (TBS-T) supplemented with 5% skim milk powder. Membranes were probed overnight at 4 °C with antibodies directed against: DICER (1:200, H-212; Santa Cruz Biotechnology), CA9 (1:1,000, M75; gift from Dr Silvia Pastorekova), H3K27me3 (1:20,000, 07-449; Upstate), H3 (1:5,000, D1H2; Cell Signaling Technology), E-cadherin (1:1,000, Cell Signaling Technology), Vimentin (1:500, clone V9; Sigma), β-tubulin (1:20,000, Abcam), β-actin (1:20,000, Sigma) or eIF4E (1:1,000, BD Transduction Laboratories). Bound antibodies were visualized using horseradish peroxidase-linked secondary antibodies (GE Healthcare) and ECL luminescence (Pierce). Luciferase reporter assay A 2.5-kb fragment from the 5′-flanking region of the DICER1 gene was previously described [15] . MCF7 cells were transiently co-transfected with the DICER or CA9 promoter [70] constructs and pcDNALacZ using Lipofectamine (Invitrogen). Transfected cells were subcultured 16 h post transfection, exposed to hypoxia and finally harvested 48 h after transfection. Luciferase and β-galactosidase activity was measured using a commercial kit (Applied Biosystems) and measured on the Fluorstar Optima plate reader (BMG Labtech). Plasmids and viral infections Knockdown was achieved using lentiviral shRNA constructs directed against DICER: TRCN0000004386, TRCN000000439; HIF-1α: TRCN0000003810; KDM6A: TRCN0000107760; KDM6B: TRCN0000236677; green fluorescent protein as control: TRCN0000072181. DICER open reading frame was cloned into pLenti CMV DEST using Gateway LR Clonase II (Invitrogen). Pri-miR200b was cloned into pLJM1 as Age 1/ Eco R1 fragment. Lentiviral particles were generated by co-transfection of 293T cells with packaging plasmids pCMVdR8.74psPAX2 and pMD2.G, together with shRNA vector pLKO.1 using Lipofectamine 2000. Virus supernatant was harvested 48 and 72 h post transfection. Cell lines were transduced with lentiviral supernatant in the presence of 8 μg ml −1 polybrene. Infected cells were selected for 48 h in 2 μg ml −1 puromycin-containing media or 7 days in 5 μg ml −1 blasticidin-containing media. Validated siRNA duplexes directed against EZH2 (ref. 52 ) 5′- AAGACTCTGAATGCAGTTGCT -3′ and HIF1α 5′- CUGAUGACCAGCAACUUGA -3′ were ordered from Sigma. Stealth RNA interference-negative control was ordered from Invitrogen (12935-300). For siRNA experiments, cells were transfected 72 h before analysis with 2 nM siRNA duplex using Lipofectamine (Invitrogen). Chromatin immunoprecipitation MCF7 and HMLER cells were fixed in 1% formaldehyde. Cross-linking was allowed to proceed for 10 min at room temperature and stopped by addition of glycine at a final concentration of 0.125 M, followed by an additional incubation for 5 min. Fixed cells were washed twice with PBS and harvested in SDS buffer (50 mM Tris at pH 8.1, 0.5% SDS, 100 mM NaCl, 5 mM EDTA), supplemented with protease inhibitors (Aprotinin, Antipain and Leupeptin all at 5 μg ml −1 and 1 mM phenylmethylsulfonyl fluoride). Cells were pelleted by centrifugation and suspended in IP Buffer (100 mM Tris at pH 8.6, 100 mM NaCl, 0.3% SDS, 1.7% Triton X-100 and 5 mM EDTA), containing protease inhibitors. Cells were disrupted by sonication, yielding genomic DNA fragments with a bulk size of 200–500 bp. For each immunoprecipitation, 1 ml of lysate was precleared by addition of 35 μl of blocked protein A beads (50% slurry protein A-Sepharose (Amersham); 0.5 mg ml −1 fatty acid-free BSA (Sigma); and 0.2 mg ml −1 herring sperm DNA in TE), followed by clarification by centrifugation. Ten-microlitre aliquots of precleared suspension were reserved as input DNA and kept at 4 °C. Samples were immunoprecipitated overnight at 4 °C using 1 μg of antibodies for either HA as a negative control (sc-805; Santa Cruz), H3K27me3 (07-449; Upstate), EZH2 (AC22, Millipore), KDM6A (ab36938, Abcam) or KDM6B (ab85392, Abcam). Immune complexes were recovered by adding 40 μl of blocked protein A beads and incubated for 4 h at 4 °C. Beads were washed three times in 1 ml of Mixed Micelle Buffer (20 mM Tris at pH 8.1, 150 mM NaCl, 5 mM EDTA, 5% w/v sucrose, 1% Triton X-100 and 0.2% SDS), twice in 1 ml of Buffer 500 (50 mM HEPES at pH 7.5, 0.1% w/v deoxycholic acid, 1% Triton X-100 and 1 mM EDTA), twice in 1 ml of LiCl Detergent Wash Buffer (10 mM Tris at pH 8.0, 0.5% deoxycholic acid, 0.5% NP-40, 250 mM LiCl and 1 mM EDTA) and once in 1 ml of TE. Immunocomplexes were eluted from beads in 250 μl elution buffer (1% SDS and 0.1 M NaHCO 3 ) for 2 h at 65 °C with continuous shaking at 1,000 r.p.m., and after centrifugation supernatants were collected. Two hundred and fifty microlitres elution buffer was added to input DNA samples and these were processed in parallel with eluted samples. Cross-links were reversed overnight at 65 °C followed by a 2-h digestion with RNAseA at 37 °C and 2 h proteinase K (0.2 μg ml −1 ) at 55 °C. DNA fragments were recovered using QIAquick PCR purification columns, according to manufacturers’ instructions. Samples were eluted in 75 μl EB buffer and then further 1/5 diluted in TE buffer. The immunoprecipitated DNA was quantified by real-time qPCR using SYBR Green I (Applied Biosystems) and following forward and reverse primers: DICER: F-5′- CGGTGGGCGTTAAATAAGTG -3′ and R-5′- CCCCCATACTGAGATGCTGT -3′. After PCR, melting curves were acquired to ensure that a single product was amplified in the reaction. Global miRNA profiling Total RNA was isolated from cells bearing shDICER G6 and pLKO.1 as control or cells exposed to hypoxia, and samples were subjected to Nanostring analysis using the Nanostring Human v2 miRNA code set at the UHN Microarray Centre. miRNAs with counts equal or lower than the negative controls were discarded from the analysis. miRNA counts were normalized to housekeeping gene RPLP0 and averaged for three independent experiments. Fluorescence-activated cell sorting FACS analysis was performed on a BD FACS Calibur (Becton Dickinson) using PE-conjugated anti-CD24 antibody (clone ML5) and APC-conjugated anti-CD44 (clone G44-26) (BD Bioscience). Mammosphere culture Mammosphere culture was performed as previously described [71] , with slight modifications. The mammospheres were cultured for 7–10 days in MammoCult media (StemCell Technologies) supplemented with 4 μg ml −1 heparin (Sigma) and 0.5 μg ml −1 hydrocortisone (Sigma). For sphere formation assays, mammospheres were dissociated to single cells with trypsin and 500 dissociated cells were plated in a 96-well plate and cultured for 10 days. Mammospheres with diameter >75 μm were counted. In vivo models All animal experiments were performed under protocols approved by the Ontario Cancer Institute’s Animal Care Committee, according the regulations of the Canadian Council on Animal Care. Female NOD-SCID mice at 6–8 weeks old were used to inject HMLER cells into the inguinal mammary fat pad (1 × 10 6 cells in a 1:1 mixture of BD Matrigel and media) following anaesthetization with isoflurane. One week before the injection of cells, a 60-day release pellet containing 2 mg 17β-estradiol and 20 mg progesterone (Innovative Research of America) was implanted subcutaneously into each mouse. At end point, mice were sacrificed, tumours harvested and optical coherence tomography embedded for immunohistochemical staining and analysis. Immunohistochemical staining and image analysis The expression of CD44 and EF5 in orthotopic xenografts was investigated as follows: Flash-frozen tissue samples were embedded in optical coherence tomography and stored at −80 °C until sectioned. Sections were thawed at room temperature before fixation in 2% paraformaldehyde for 20 min. After washing sections in PBS, sections were permeabilized in PBS containing 0.5% Triton X-100 for 15 min, wash 3 × 5 min in PBS-T and then incubated in a primary antibody cocktail of mouse anti-human CD44 (1:75, BD Pharmingen) and rat anti-mouse CD31 (1:300, BD Pharmingen) or anti-human H3K27me3 (1:500, C36B11; Cell Signalling) overnight at room temperature. Sections were subsequently washed 3 × 5 min in PBS-T followed by incubation in a secondary antibody cocktail of goat anti-mouse Alexafluor 488 (1:200, Life Technologies) and goat anti-rat Alexafluor 555 (1:200, Life technologies) or goat anti-mouse Alexafluor 488 (1:200, Life Technologies) for 1 h at room temperature. After washing in PBS-T, sections were incubated in EF5-Cy5 (1:50, provided by Dr Cameron Koch) for 3 h at room temperature. After washing, sections were finally incubated in a working solution of DAPI (4',6-diamidino-2-phenylindole) for 5 min, washed, dried and imaged on a laser scanning microscope (Huron Technologies). Images were analysed using Definiens Tissue Studio software, which allows for semi-automatic histology image analysis. Briefly, the software was trained to identify viable tumour areas, necrotic areas, tumour stroma and empty areas within the scanned section. A threshold was determined by mean +2 s.d. intensity in the EF5 and CD44 channels. The average CD44 staining intensity within the tumour area was measured in both EF5-negative and -positive areas. EF5-positive area above a background threshold was obtained from the average intensity of all tumour sections. Statistical analyses Unless otherwise stated, a Student’s t -test or one-way analysis of variance with Bonferroni’s post-hoc test were used to test significance between populations. A significance threshold of P <0.05 was applied. Points and error bars plotted in graphs represent the mean±s.e.m for three or more independent experiments. How to cite this article: van den Beucken, T. et al . Hypoxia promotes stem cell phenotypes and poor prognosis through epigenetic regulation of DICER. Nat. Commun. 5:5203 doi: 10.1038/ncomms6203 (2014). Accessions codes: miRNA profiling and ChIP-Seq data have been deposited in the NCBI Gene Expression Omnibus database under accession codes GSE61722 and GSE61740 , respectively.